Topological superconductivity and unconventional pairing in oxide interfaces Pinpointing the microscopic mechanism for superconductivity has proven to be one of the most outstanding challenges in the physics of correlated quantum matter. Thus far, the most direct evidence for an electronic pairing mechanism is the observation of a new symmetry of the order parameter, as done in the cuprate high-temperature superconductors. Alternatively, global, topological invariants allow for a sharp discrimination between states of matter that cannot be transformed into each other adiabatically. Here we propose an unconventional pairing state for the electron fluid in two-dimensional oxide interfaces and establish a direct link to the emergence of non-trivial topological invariants. Topological signatures, in particular Majorana edge states, can then be used to detect the microscopic origin of superconductivity. In addition, we show that also the density wave states that compete with superconductivity sensitively depend on the nature of the pairing interaction. The two-dimensional (2D) electron fluid that forms [1] at the interface between the insulators SrTiO 3 and LaAlO 3 is an example of an engineered quantum system, where a new state of matter emerges as one combines the appropriate building blocks. The subsequent discovery of superconductivity [2] in the interface, along with the ability to control the ground state via applied electric fields [3] opened up intense research. The key open question is whether electronic correlations promote novel phases, such as unconventional superconductivity or exotic magnetically ordered states [4] , [5] , [6] , [7] , [8] and how such phases are related to each other. Generally speaking, new states of matter can be sharply distinguished from conventional behaviour when they break a symmetry or differ in their topology. An example for the former case are the cuprate high-temperature superconductors [9] , [10] . The second category consists of topological insulators and superconductors, which have recently had a major impact on solid state physics [11] , [12] . Here the Bloch Hamiltonian, a mapping from momentum space to the space of Hamiltonians, is not adiabatically connected to the vacuum. In this paper, we establish a direct connection between pairing mechanism and topology of the superconducting state at the interface: Unconventional pairing, that is superconductivity based on the exchange of particle–hole excitations, leads to a topological phase with Majorana bound states and related non-trivial topological aspects. More specifically, we find a time-reversal preserving topological superconductor that has attracted recent attention [13] , [14] , [15] , [16] , [17] , [18] . In contrast, conventional electron–phonon coupling in the same system would yield a topologically trivial state. Consequently, our results allow to identify the unresolved microscopic mechanism of superconductivity in oxide interfaces by probing the topological properties of the pairing state. We also study competing phases, expected to emerge nearby superconductivity in the phase diagram. For a conventional pairing mechanism we find charge density wave order, while an in-plane spin density wave with magnetic vortices competes with unconventional superconductivity. Interacting low-energy model It is well known that the relevant low-energy degrees of freedom at the interface are made up of the titanium 3 d xy , 3 d xz and 3 d yz orbitals [19] , [20] . There has been an ongoing debate about why the concentration of transport carriers is considerably lower than what is seen in local charge measurements or expected from the polar catastrophe. One widely accepted explanation [21] , [22] , [23] is that the electrons in the 3 d xy states, that are spatially much closer to the interface than the other orbitals, are mainly localized, whereas the electrons occupying the 3 d xz and 3 d yz orbitals are delocalized. It indicates that the key electrons at the interface, at least for understanding superconductivity, reside in the 3 d xz and 3 d yz states. This picture is confirmed by the experimental observation that the emergence of superconductivity is correlated with the chemical potential entering the 3 d xz and 3 d yz orbitals [24] , [25] . Thus, we assume that the crucial states near the Fermi energy of the oxide interface are made up of titanium 3 d xz and 3 d yz orbitals. The orientation of the electron clouds leads to a wave function overlap along the x direction that is much larger for 3 d xz states compared with 3 d yz , and vice versa for the y direction. Each orbital is then characterized by a light mass m l and a heavy mass m h , leading to the experimentally observed strongly anisotropic electronic structure [19] , [20] . For example, the energy of the 3 d xz states can be described by where m h / m l ≃ 15…30. ε yz follows from equation (1) by interchanging k x and k y . In addition, the electronic properties of the polar interface between insulating oxides is strongly affected by the spin–orbit interaction. Due to the Dresselhaus–Rashba effect [26] , [27] , the electronic states experience a momentum-dependent splitting and mixing of spin states, naturally explaining magnetotransport experiments [28] , [29] . The effect might also be responsible for the observed phase separation in the interfaces [30] . Focusing on the 3 d xz and 3 d yz states, the most general form up to linear order in momentum that is consistent with the C 4 ε -point-group symmetry and time-reversal invariance is given by where the Pauli matrices σ i and τ j ( i , j =0…3) act in spin and orbital space, respectively. To determine the coefficients α i in equation (2), we performed a microscopic calculation (see Supplementary Methods ) first including the 3 d xy orbital together with the atomic spin–orbit coupling and the hopping matrix elements i δ k y ( i δ k x ) between the 3 d xy and 3 d xz (3 d yz ) orbitals along the y axis ( x axis). The amplitude δ , which can only be finite as the inversion symmetry is broken, has been shown in ref. 31 , to be an essential ingredient for understanding the band structure of the interface electron system. Despite being shifted down in energy by ε 0 , we can project out the 3 d xy band due to the spatial separation of the 3 d xy and 3 d xz (3 d yz ) orbitals. This yields the spin–orbit coupling in equation (2) with . The values λ ≃ 20 meV, δ / a 0 ≃ 40 meV with a 0 denoting the in-plane lattice constant, and ε 0 ≃ 250 meV were determined in first principles calculations [31] . As δ and ε 0 depend sensitively on details of the interface we use α 0 ≃ 10…50 meVÅ, estimated from magnetotransport experiments [28] . In Fig. 1a the bands that result from the combination of the anisotropic masses in equation (1) and the spin–orbit coupling in equation (2) are shown. Two of the four bands are pushed to higher energies by the atomic spin–orbit coupling λτ 2 σ 3 and can thus be neglected for the following low-energy analysis as long as the chemical potential is tuned sufficiently far away from the bottom of these bands. The remaining two bands are split by the Dresselhaus–Rashba coupling and show strong nesting in the highlighted regions. The nesting is a consequence of the mass anisotropy and becomes exact in the limit m l / m h →0. 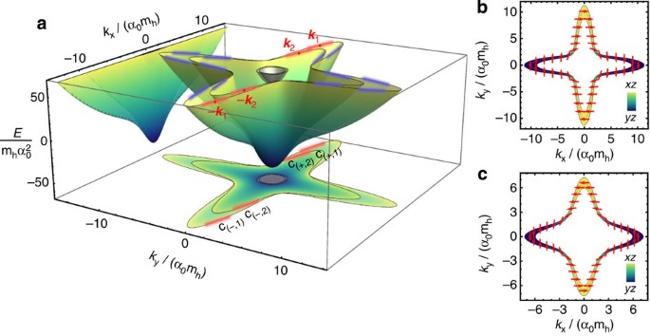Figure 1: The bands and the wave functions of our model. (a) The spectrum of the effective two-orbital Hamiltonian using the realistic parameters stated in the main text. In this paper, we restrict the analysis on the four most strongly nested subspaces (highlighted in red and blue). The orbital weight (colour) and orientation of the spin (red arrows) are illustrated in (b) and (c) for the outer and inner Fermi surface, respectively. Note that, as a consequence of time reversal and π-rotation symmetry about thezaxis, the spin has to lie in thexyplane. Figure 1: The bands and the wave functions of our model. ( a ) The spectrum of the effective two-orbital Hamiltonian using the realistic parameters stated in the main text. In this paper, we restrict the analysis on the four most strongly nested subspaces (highlighted in red and blue). The orbital weight (colour) and orientation of the spin (red arrows) are illustrated in ( b ) and ( c ) for the outer and inner Fermi surface, respectively. Note that, as a consequence of time reversal and π-rotation symmetry about the z axis, the spin has to lie in the xy plane. Full size image This allows us to use a low-energy theory that involves only the degrees of freedom in the vicinity of the most parallel slices of the Fermi surface. In total, there are four equivalent strongly nested subspaces that are related by the point-group symmetries. Without loss of generality, let us focus on the one indicated in red in Fig. 1a . In this subset of momentum space, we introduce helicity annihilation and creation operators c ( σ , j ) and that diagonalize the quadratic part of the Hamiltonian. Here σ =± refers to the sign of k x and j =1 ( j =2) denotes the outer (inner) Fermi surface. To relate these operators to observables, Figs 1b,c show the spin orientation and the orbital weight of the states in the vicinity of the outer and inner Fermi surface, respectively. We emphasize the similarity of both the form of the Fermi surface and the spin/orbital textures to the results reported in ref. 20 for the surface states of SrTiO 3 . There are two types of interaction processes allowed by momentum conservation, which we will refer to as backscattering and forward scattering. The most general momentum-independent backscattering term is given by where ( σ =±) From now on, the Pauli matrices σ s , as in equation (4), do not describe the physical spin, but rather act in the abstract isospin space of the local helicity operators. The momentum of the operator c ( σ , j ) is measured relative to the centre σ k j of the corresponding red region in Fig. 1a . Using the phase convention for the eigenstates defined in the Methods, one finds that the π -rotation symmetry with respect to the z axis implies that u has to be symmetric, u T = u . The remaining symmetries of the point group then fully determine the interaction in the other three most strongly nested subspaces. In addition, time-reversal symmetry imposes the constraint if either s =2 or . Let us first assume that the cut-off for the momenta perpendicular to the Fermi surface can be chosen smaller than the distance between the inner and outer Fermi surface (below we will also discuss the opposite limit of nearly degenerate Fermi surfaces). This means that the red regions in Fig. 1a do not overlap. In this situation, momentum conservation rules out further interaction processes such that only u 00 , u 11 =− u 22 , u 33 and u 30 = u 03 can be non-zero. As the notation in equation (3) is rather abstract, we represent the four allowed backscattering terms in Figs 2a–d graphically in the helicity basis. One finds two distinct intraband Coulomb terms ( U 1 , U 2 ), interband Coloumb interaction ( U ′) as well as pair hopping ( J ). 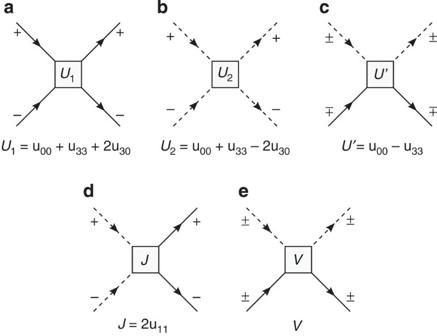Figure 2: Diagrammatic representation of the scattering processes. In case of strong spin–orbit coupling, the combination of momentum conservation, time reversal and rotation symmetry allow for four independent backscattering processes (a–d) and one forward scattering term (e). Solid and dashed lines refer to the outer and inner Fermi surface and ± indicates the sign ofkxin the four red regions ofFig. 1a. Figure 2: Diagrammatic representation of the scattering processes. In case of strong spin–orbit coupling, the combination of momentum conservation, time reversal and rotation symmetry allow for four independent backscattering processes ( a – d ) and one forward scattering term ( e ). Solid and dashed lines refer to the outer and inner Fermi surface and ± indicates the sign of k x in the four red regions of Fig. 1a . Full size image In case of forward scattering, where all four fermions have the same index σ , the combination of Fermi statistics and point symmetries leads to only one independent coupling constant. The associated process ( V ) is illustrated in Fig. 2e . Pairing instabilities Having derived the interacting low-energy Hamiltonian, we can now deduce the associated instabilities. We perform a standard fermionic one-loop Wilson renormalization group (RG) calculation [32] , in which high-energy degrees of freedom are successively integrated out yielding an effective Hamiltonian with renormalized coupling constants. If, during this procedure, some of the couplings diverge, the system will develop an instability. Following refs 33 , 34 we identify the physical nature of this instability by determining the order parameter that has the highest transition temperature, allowing for all possible (momentum independent) particle–hole and particle–particle ordered states: where α and β are double indices comprising helicity σ =± and the Fermi surface sheet index j =1,2. Near the Fermi surface, we linearize the band dispersion ε ( k ) ≃ ± ε j k ⊥ with k ⊥ denoting the component of the momentum perpendicular to the Fermi surface. For simplicity, let us first focus on the situation ε 1 = ε 2 , which is quantitatively a good approximation even when the chemical potential gets closer to the bottom of these bands. Below, we will also investigate the more general case ε 1 ≠ ε 2 . If ε 1 = ε 2 , only u 11 and u 33 out of the five coupling constants flow. In the associated flow diagram in Fig. 3a , we find two regimes, denoted by (I) and (II), where the running couplings diverge. Using the notation of Fig. 2 , it holds − U 1 ~ − U 2 ~ U ′~ ± J /2 ≫ | V |, U ′>0, at the associated strong coupling fixed points with + and − referring to regime (I) and (II), respectively. In both cases, the instability is of superconducting type characterized by the two non-zero anomalous expectation values , j =1,2, having equal modulus. As expected, there is only intra-Fermi surface pairing, implying that only Kramers partners are paired. In region (I), the superconducting order parameters of the nearby Fermi surfaces have opposite sign, whereas in (II) the sign is the same. The corresponding superconducting states will be denoted by SC +− and SC ++ , respectively. Rewriting the order parameters in the spin basis, one finds a mixture of singlet and triplet pairing, where both components are of equal strength in the strongly nested domains and the triplet pairing vector points perpendicular to the Fermi surface. 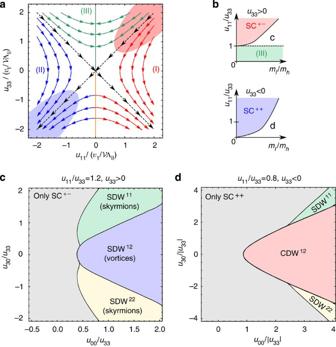Figure 3: RG flow and the resulting phase diagrams. (a) The flow of the two running coupling constants in the case of identical Fermi velocities is shown. Hereand Λdenote the volume of the system and the cut-off of the nested subspaces tangential to the Fermi surface. Only in the regimes (I) and (II) the couplings diverge indicating that the system develops an instability. The red (blue) region corresponds to the bare couplings for a microscopically repulsive (attractive) interaction. The schematic phase diagrams taking into account finite mass anisotropies are shown in part (b). The non-flowing couplings determine the properties of the charge density wave as shown in (c) and (d) for the unconventional and conventional superconductor, respectively. The nomenclature of the phases is explained in the main text. Figure 3: RG flow and the resulting phase diagrams. ( a ) The flow of the two running coupling constants in the case of identical Fermi velocities is shown. Here and Λ denote the volume of the system and the cut-off of the nested subspaces tangential to the Fermi surface. Only in the regimes (I) and (II) the couplings diverge indicating that the system develops an instability. The red (blue) region corresponds to the bare couplings for a microscopically repulsive (attractive) interaction. The schematic phase diagrams taking into account finite mass anisotropies are shown in part ( b ). The non-flowing couplings determine the properties of the charge density wave as shown in ( c ) and ( d ) for the unconventional and conventional superconductor, respectively. The nomenclature of the phases is explained in the main text. Full size image In the region (III), none of the coupling constants diverge, which means that for sufficiently small bare couplings the system will not develop any instability and, thus, reside in the metallic phase. To unveil the microscopic pairing mechanism of the two superconducting states, we start from a repulsive Coulomb interaction between the 3 d orbitals and project onto the effective low-energy theory. This places us into region (I) of the RG flow in Fig. 3a . In contrast, an attractive interaction due to electron–phonon coupling would lead to initial couplings in region (II). Consequently, SC ++ results from conventional electron–phonon pairing, whereas SC +− is an unconventional superconductor, where particle–hole fluctuations effectively change the sign of u 33 . Topological superconductivity Both SC +− and SC ++ respect time-reversal symmetry as far as the degrees of freedom of the nested subspaces are concerned. It is natural to assume that this holds for the entire Fermi surface and that, in addition, the system does not break the point symmetries relating the nested segments. In this case the gap is finite on the entire Fermi surface as seen in recent experiments [35] . Being fully gapped, it is obvious to ask whether the time-reversal invariant 2D superconductor (class [36] DIII) is topologically trivial or non-trivial [37] , which is of great interest as it strongly influences its physical properties. The most prominent feature of a non-trivial topological superconductor is the appearance of spin-filtered counter propagating Majorana modes at its edge when surrounded by a trivial phase [38] . It has been shown [39] that, in the weak-pairing limit, the associated topological invariant is fully determined by the sign of the paring field on the Fermi surfaces. For non-degenerate Fermi surfaces, it holds where the product involves all Fermi surfaces, and Δ j denote the wave function of the non-interacting part of the Hamiltonian and the pairing field at an arbitrary point on the j th Fermi surface. Furthermore, m j is the number of time-reversal invariant points enclosed by the j th Fermi surface and T is the unitary part of the time-reversal operator, given by T = iτ 0 σ y in the basis of equation (2). As, in the present case, both Fermi surfaces enclose only one time-reversal invariant point, the superconductor is topological (trivial) if the sign of δ j is different (identical) on the two Fermi surfaces. Note that no additional Fermi surfaces are introduced when the continuum description of the theory is replaced by the properly lattice periodic tight-binding Hamiltonian. This is important as topological band theory is only well defined for lattice periodic systems. Inserting the order parameters derived above, we obtain the pairing Hamiltonian with , for the superconductor SC ++ and , for the SC +− state. Calculating δ j in equation (6), one finds (see Methods for more details) that the superconductor is topological if and trivial for the reversed inequality sign. At , the gap closes as is characteristic for a topological phase transition. Recalling the flow depicted in Fig. 3a , one immediately sees that SC ++ is trivial, whereas SC +− is a topological superconductor. Accordingly, the experimental observation of topological features of the superconducting state implies that the pairing mechanism must be unconventional as it is the case for SC +− . Vice versa, a trivial state is only consistent with conventional, electron–phonon induced superconductivity. Note that the pairing states obtained here differ from the results of former studies [40] , [41] , [42] of interacting single-band models with Rashba spin–orbit coupling for the following reasons: The anisotropic masses lead to strong nesting, the inclusion of two orbitals allows both for more independent interaction terms and for additional spin–orbit couplings that crucially affect the spin textures. Furthermore, we emphasize the difference of our result to recent work [43] , [44] , [45] , [46] proposing the emergence of Majorana fermions in the heterostructure as a consequence of the coexistence of magnetism and superconductivity. In that case, however, (physical, spin-1/2) time-reversal symmetry is broken, whereas the SC +− state found here is time-reversal invariant. Competing phases and spin textures Eventually, our RG flow will always favour a superconducting state. However, by successively reducing the characteristic energy scale, we are increasingly sensitive to details of the low-energy theory and, consequently, the fact that the nesting is not perfect becomes relevant. For any finite m l / m h , the strongly nested domains of the Fermi surface have a non-vanishing curvature, thus, eventually forcing the RG flow to stop. If the flow is terminated before any of the coupling constants diverges, other phases competing with superconductivity can emerge, as illustrated in Fig. 3b . In the associated mean-field equations, all coupling constants can now be of the same order and, hence, the resulting diagram of competing phases depends on all couplings, also on those that do not flow. The analysis yields that either a charge density wave (CDW 12 ) or three different spin density waves (SDW 11 , SDW 22 , SDW 12 ) are possible or the corresponding superconducting states are dominant for arbitrary m l / m h as shown in Fig. 3c,d . The superscripts in the density waves CDW ij and SDW ij refer to the particle–hole expectation value (and i ↔ j , if i ≠ j ) that is non-zero in the respective phase. The difference between CDW 12 and SDW 12 is the relative sign of and , rendering the order parameter symmetric and antisymmetric under time reversal in the former and in the latter case, respectively. The spatial structure of the charge and spin density waves can easily be determined from the wave functions of the system and the order parameters . In analogy to the discussion of the superconducting states, we assume that no additional point-group symmetry is broken. In the case of the CDW 12 phase, one then finds that the local charge density is given by where Q 12 = k 1 + k 2 is the associated nesting vector. The first contribution stems solely from the nested subspace highlighted in red in Fig. 1a and the ellipsis stands for the terms emanating from the remaining three subspaces, which are fully determined by the π/2 rotation and reflection symmetry at the xz plane. The resulting charge profile is illustrated in Fig. 4a . Note that the periodicity crucially depends on the ratio of the x and y component of the nesting vector Q 12 . 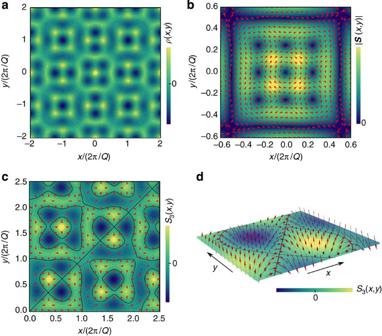Figure 4: The spatial structure of the different density wave phases. (a) The charge density pattern of CDW12. In SDW12, where the nesting vector is again given byQ12=k1+k2, the spinSlies approximately in thexyplane. As shown in (b) using red arrows to indicate the direction of the spin, one finds a lattice of vortices. In case of SDW11, the nesting vector is 2k1and we observe a lattice of skyrmions and antiskyrmions as illustrated in (c), where the red arrows indicate the direction of thexycomponents of the spin and the black lines are the zeros of itszcomponentS3. (d) One of the emerging closely bound skyrmion–antiskyrmion pairs. The texture of SDW22(nesting vector 2k2) is identical to SDW11up on replacingS3→−S3. In all plots, a nesting vector of the form (2, 0.48)Qhas been assumed. Figure 4: The spatial structure of the different density wave phases. ( a ) The charge density pattern of CDW 12 . In SDW 12 , where the nesting vector is again given by Q 12 = k 1 + k 2 , the spin S lies approximately in the xy plane. As shown in ( b ) using red arrows to indicate the direction of the spin, one finds a lattice of vortices. In case of SDW 11 , the nesting vector is 2 k 1 and we observe a lattice of skyrmions and antiskyrmions as illustrated in ( c ), where the red arrows indicate the direction of the xy components of the spin and the black lines are the zeros of its z component S 3 . ( d ) One of the emerging closely bound skyrmion–antiskyrmion pairs. The texture of SDW 22 (nesting vector 2 k 2 ) is identical to SDW 11 up on replacing S 3 →− S 3 . In all plots, a nesting vector of the form (2, 0.48) Q has been assumed. Full size image Similarly, the spatial structure of the spin density waves SDW 12 and SDW 11 , SDW 22 can be calculated (for details see Supplementary Methods ) yielding the textures shown in Fig. 4b and Fig. 4c , respectively. Here we have used that, in the red regions of Fig. 1a , the spins are approximately aligned along the y axis (see Fig. 1b,c ). Within this approximation, the expectation value of the spin lies in the xy plane in case of the spin density phase SDW 12 . The 2D vector field is a lattice of vortices, both with positive and negative winding numbers. In the phases SDW 11 and SDW 22 , the spin is free to rotate in three dimensions. One finds a complicated periodic arrangement of isolated skyrmions and antiskyrmions, as well as closely bound skyrmion–antiskyrmion pairs (see Fig. 4d ). The emergence of a skyrmion lattice that leads to interesting physical effects (see for example ref. 47 ), is consistent with recent work [8] , [48] pointing out that these magnetic topological defects naturally appear as solutions of the Ginzburg–Landau equations for systems with spin–orbit interaction. On top of that, the difference between the density wave phases in Figs 3c,d neighbouring the superconducting states SC +− and SC ++ can be exploited to gain information about the pairing mechanism in the heterostructure. As the orbital contribution to the magnetization is negligible for large mass anisotropies, the experimental observation of in-plane magnetization [5] is only consistent with the SDW 12 state. This implies that the superconducting phase of SrTiO 3 /LaAlO 3 is supposed to be unconventional and topologically non-trivial. As the Z 2 invariant N is a rather abstract way of classifying superconducting phases, it is worthwhile to gain intuitive understanding for why identical (different) signs of the pairing fields lead to a topologically trivial (non-trivial) superconductor. Imagine starting from the standard s -wave singlet BCS superconductor, characterized by an isotropic, spin-degenerate Fermi surface, where only Kramers partners are paired. Turning on terms that break inversion and rotation symmetry, this phase can be continuously deformed into the SC ++ state without closing the gap as illustrated in Fig. 5 . This proves that the SC ++ phase is, exactly as the BCS superconductor, topologically trivial. Importantly, relative phases between the pairing fields of the two Fermi surfaces cannot be introduced adiabatically without breaking time-reversal symmetry. Therefore, deforming the BCS state continuously into the SC +− superconductor necessarily involves a closing of the gap on one of the Fermi surfaces. At this gap closing, a topological phase transition occurs as we have shown mathematically by calculating the invariant N for the SC +− state. Note that a similar topological phase has been found very recently in a prototype model of 2D 3 He-B with the assumption of Rashba spin–orbit coupling [49] . 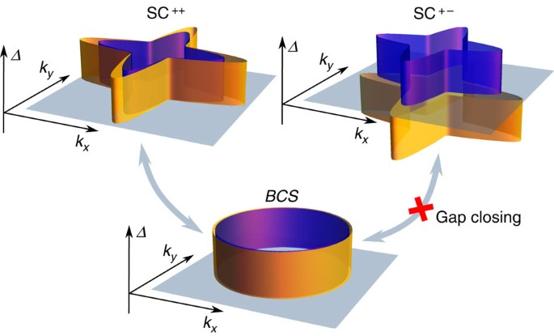Figure 5: Illustration of the topological properties. The value of the pairing field at the inner (blue) and outer (orange) Fermi surface is shown for thes-wave singlet BCS superconductor as well as for the SC++/SC+−phases. The topologically trivial BCS state is adiabatically connected to the SC++superconductor, whereas a continuous deformation into the SC+−phase requires closing the gap at some point along the path. Figure 5: Illustration of the topological properties. The value of the pairing field at the inner (blue) and outer (orange) Fermi surface is shown for the s -wave singlet BCS superconductor as well as for the SC ++ /SC +− phases. The topologically trivial BCS state is adiabatically connected to the SC ++ superconductor, whereas a continuous deformation into the SC +− phase requires closing the gap at some point along the path. Full size image Our link between topology and pairing mechanism allows to unveil the unknown microscopic physics of the superconductor by observing signatures of Majorana bound states: In case of the unconventional SC +− state, counter propagating Majorana modes are expected to be localized on a length scale of the order of the coherence length [2] ξ ≃ 100 nm at boundaries to trivially gapped phases. These modes can be probed experimentally, for example, using tunnel spectroscopy or via thermal conductivity measurements [50] . From the material science point of view, it is important to distinguish between ‘intrinsic’ and ‘extrinsic’ topological superconductors. In ‘extrinsic’ systems (see, for example, refs 16 , 17 , 18 ) Cooper pairs are injected via the proximity effect from a non-topological superconductor into another conductor that is thereby driven into a topological superconducting phase. The SC +− state is an ‘intrinsic’ topological superconductor, where the pairing and the non-trivial topology emerges from the material’s internal dynamics, which could simplify probing Majorana physics. One additional advantage of oxide interfaces for investigating Majorana modes is that boundaries of highly controllable shape between superconducting and insulating phases can be realized experimentally, either via locally reducing the thickness of the LaAlO 3 crystal [51] or using a voltage-biased atomic force microscope tip [52] . As already stated above, we have also considered the case of different Fermi velocities, ε 1 ≠ ε 2 (see Supplementary Note 1 for more details of the analysis). Then all four backscattering couplings, the interaction terms in Figs 2a–d , flow. Nonetheless, exactly as before, the leading instability is generically superconducting for sufficiently large mass anisotropies. Detuning the Fermi velocities leads to a crossover from the superconductors SC +− and SC ++ , which are characterized by , to a pairing state where the anomalous expectation value is only finite on the Fermi surface with the larger Fermi velocity. Note that, in this limit, the associated mean-field Hamiltonian still describes pairing on both Fermi surfaces due to the pair hopping term, giving rise to a fully gapped phase. Remarkably, we again find that the superconductor resulting from the conventional electron–phonon pairing mechanism is topologically trivial, whereas the unconventional superconductor is non-trivial. This proves that the correspondence between the pairing mechanism and the topological properties of the superconducting phases in the heterostructure holds irrespective of the values of the Fermi velocities. For completeness, we have also investigated the case of very weak spin–orbit interaction where the energetic cut-off of the low-energy model is much larger than the spin–orbit splitting (see Supplementary Note 2 ). Then the red regions in Fig. 1a merge pairwise and, consequently, momentum conservation is much less restrictive making more backscattering terms possible. Surprisingly, even in this situation, the observation of a topologically non-trivial superconducting phase is only consistent with the pairing mechanism being unconventional. Finally, we point out that the pairing state of a many-body system is always a consequence of the combination of electron–phonon and electron–electron interactions. Even if phonons enhance a sign-changing pairing state, the electron–phonon coupling alone prefers quite generally conventional pairing (see, for example, refs 53 , 54 , 55 ). This includes the recently proposed scenario, where odd-parity pairing states and related topological superconductivity [13] are predicted to occur in systems with an electron–phonon coupling that is singular at long wavelength and closely tied to inversion symmetry [56] , [57] . The interesting mechanism of refs 56 , 57 does not apply to the oxide interfaces studied here, as inversion symmetry is broken, the transferred momentum is finite, and since tunnelling data indicate a fully established superconducting gap [35] . Thus, we conclude that for the oxide interfaces the established link between topology and microscopic mechanism is robust. In summary, our analysis reveals that the phase diagram of the 2D electron fluid forming at the interface between the perovskite oxides LaAlO 3 and SrTiO 3 combines two fascinating notions of condensed matter physics: Topology and unconventional superconductivity. We find that, very generically, the observation of signatures of topologically non-trivial superconductivity, such as the appearance of Majorana bond states, directly implies that the underlying pairing mechanism must be unconventional. In addition, the spin density wave phases competing with topological superconductivity show topological spatial textures as well. Depending on the value of the coupling constants, we find lattices of both skyrmions and vortices. Phase convention for the helicity states Using a path-integral representation, the quadratic part of the theory can be written as where k ≡( ω n , k ) and Ψ, are four-component Grassmann fields describing spinful fermions in the 3 d xz and 3 d yz orbitals. Furthermore, H is the Hamiltonian defined in the main text characterized by the anisotropic masses (1) and the spin–orbit coupling in equation (2). We diagonalize S 0 by performing the unitary transformation where with φ α ( k ) denoting an eigenvector of H ( k ). As explained in the main text, we can restrict the analysis of instabilities to one of the most strongly nested subspaces and introduce helicity fields c ( σ , j ) and in the local coordinate systems yielding after linearizing the spectrum. Here s 1 =+1, s 2 =−1 and η denotes the spin–orbit splitting in the case of quasi-degenerate Fermi surfaces. For stronger spin–orbit coupling, where the four red regions in Fig. 1a are disjoint, one has η =0 by construction. The different regimes of the quasi one-dimensional description in equation (12) are summarized graphically in Supplementary Fig. 1 . In equation (12) and in the following, we use the compact notation k ≡(ω n , k ∥ , k ⊥ ) and where Λ ⊥ and Λ | are the momentum cutoffs normal and tangential to the Fermi surface. To make the helicity operators unique, we have to fix the phases of the eigenstates in equation (11). This is achieved by exploiting the invariance of the Hamiltonian under π -rotation R c 2 and time-reversal Θ. The former symmetry implies that and hence we can construct the eigenstates with negative k x from those with k x >0 via Consecutive application of time reversal and π-rotation leads to the k -space local antiunitary symmetry of the Hamiltonian. Thus, we can adjust the phases of the eigenstates such that for k x >0. From equation (15), it follows that equation (17) actually holds also for k x <0. Representation of the symmetries Having fixed the phases of the local eigenstates, the representation of time-reversal and π-rotation symmetry on the helicity fields is well defined. Note that the remaining elements of the point-group C 4 ε cannot be represented on c and as these symmetry operations act between different most strongly nested subspaces. For the very same reason, however, these symmetries are also irrelevant when deriving the most general interaction within one of the subspaces. Time reversal acts according to in the basis of equation (9). Using equations (15) and (17), one can derive the transformation behaviour in the helicity basis. Similarly, for the π-rotation symmetry, we find and the same for . Symmetry analysis of the interaction Now we will derive the most general momentum-independent interaction of the low-energy theory consistent with the symmetries of the system. Let us write where the Greek letters are double indices comprising σ =± and j =1,2. It turns out that the dimensionless parameterization, with is very convenient for the following analysis. In equation (23), we have already taken into account that only forward scattering (described by V ) and backscattering ( W ) are allowed by momentum conservation. Throughout this work, we assume that Umklapp processes are not possible. Due to Fermi statistics, the forward scattering tensors must have the form whereas the backscattering tensor has 16 degrees of freedom, which we parametrize according to Note that g ss ′ ∝ u ss ′ with u ss ′ used in the main text to define the backscattering terms. Next, let us derive the constraints resulting from π-rotation symmetry. Demanding that equation (21) be invariant under the transformation (20), we find Consequently, all forward scattering processes are characterized by one coupling constant g 0 ≡ g 0 (+)= g 0 (−). In terms of the representation in equation (25), the second constraint is equivalent to g T = g , as stated in the main text. Similarly, to make the interaction time-reversal symmetric, we require invariance of equation (21) under equations (19a,b), . Again using the parameterization in equation (23), we find that V is not further restricted, whereas the backscattering tensor has to satisfy In the equation (25), this is equivalent to demanding g ss ′ =0 if either s =2 or s ′=2 and, hence, we have If the most strongly nested subspaces are disjoint, momentum conservation rules out further interaction terms leading to the four independent backscattering couplings discussed in the main text. Microscopic interaction An important part of our analysis is the identification of the pairing mechanisms in the different superconductors. For this purpose, we include matrix elements of the electron–electron interaction between the relevant 3 d xy and 3 d yz orbitals yielding both an intra- ( ) and inter-orbital ( ) Hubbard interaction, a Hund’s coupling ( H ) term, as well as pair hopping ( ). In addition, we use and valid for the usual Coulomb interaction, but our results do not crucially depend on this assumption. Projecting the interaction onto the low-energy theory, we find, using the model defined in the main text, in case of disjoint support in momentum space. In this way, we can estimate the initial conditions for the RG flow both for a microscopically repulsive ( g 00 >0) and for an electron–phonon induced, attractive ( g 00 <0) interaction. The two scenarios correspond, respectively, to the red- and blue-shaded regions in Fig. 3a . Wilson RG In the Wilson approach, as discussed in detail for fermions with a finite Fermi surface in ref. 32 , fast modes with momenta Λ ⊥ e −Δ l < k ⊥ <Λ ⊥ , Δ l >0, are integrated out yielding, after proper rescaling, an effective action with renormalized parameters. At one-loop order and for T =0, we find that, in all three regimes considered in this work, forward scattering is not renormalized, whereas the backscattering tensor flows according to with x j := v j / v 1 . In the simplest case of strong spin–orbit coupling and ε 1 = ε 2 , equation (30) is equivalent to yielding the flow shown in Fig. 3a . Mean-field equations and instabilities As we are only interested in determining the instability with the highest transition temperature, it is justified to linearize the mean-field equations in the order parameters. Keeping only the leading terms in the physically relevant limit T ≪ ε 2 Λ ⊥ , we find and where has been introduced. In equation (32b), it has been exploited that is antisymmetric such that it is sufficient to consider ( σ α , σ β )=(−,+). We see that, both for the density wave and for the superconducting channel, solely order parameters with σ α =− σ β are relevant. In addition, only the backscattering tensor W enters, whereas forward scattering, V , does not have any role at all. Expanding the density wave order parameters, and the anomalous expectation values, in Pauli matrices we can rewrite equations (32a,b),  more explicitly. The result for strong spin–orbit coupling and identical Fermi velocities is summarized in Supplementary Table 1 . Inserting the asymptotic behaviour of the coupling constants, that is g 11 ~ − g 33 →∞ and g 11 ~ g 33 →−∞ in regime (I) and (II), respectively, one finds the superconducting phases SC +− and SC ++ discussed in the main text. To derive the competing instabilities, we have investigated the flow of all mean-field equations in Supplementary Table 1 according to equation (31) and analysed which of the order parameters is dominant before superconductivity eventually wins. Calculation of the topological invariant To obtain N in equation (6), we have to relate the effective one-dimensional theory, equations (7) and (12), to the full mean-field Hamiltonian, defined on the entire 2D Brillouin zone. For simplicity, let us focus on the case of strong spin–orbit coupling and ε 1 = ε 2 (see Supplementary Notes 1 and 2 for the other regimes of the system). Suppose that the free Hamiltonian H has been diagonalized by applying the transformation in equation (10). Here we use the convention that the eigenfunctions φ α are sorted for every k such that the energy increases with α . From equation (7), we know that the pairing term, that is the second line in equation (36), must have the form Here S j denotes the strongly nested domain in the vicinity of k j (see red regions in Fig. 1a ). The ellipsis in equation (37) stands for the pairing terms in the remainder of the Brillouin zone. Using equation (10) to rewrite the f -operators in terms of the fields, we find By construction, H is time-reversal invariant, which means that with denoting complex conjugation and arbitrary . It is straightforward to show that time-reversal invariance of the pairing term is equivalent to Using the phase conventions in equations (15) and (17) and writing Δ 0 =|Δ 0 |e i ρ , , one finds that equation (40) is satisfied if The matrix elements where q j is an arbitrary point on the j th Fermi surface, can now be readily evaluated. Choosing q j = k j , one finds again exploiting equations (15) and (17) as well as, in the last line, equation (41). The invariant is thus given by How to cite this article: Scheurer, M. S. et al . Topological superconductivity and unconventional pairing in oxide interfaces. Nat. Commun. 6:6005 doi: 10.1038/ncomms7005 (2015).